Cell type-specific plasticity of striatal projection neurons in parkinsonism and L-DOPA-induced dyskinesia The striatum is widely viewed as the fulcrum of pathophysiology in Parkinson’s disease (PD) and L-DOPA-induced dyskinesia (LID). In these disease states, the balance in activity of striatal direct pathway spiny projection neurons (dSPNs) and indirect pathway spiny projection neurons (iSPNs) is disrupted, leading to aberrant action selection. However, it is unclear whether countervailing mechanisms are engaged in these states. Here we report that iSPN intrinsic excitability and excitatory corticostriatal synaptic connectivity were lower in PD models than normal; L-DOPA treatment restored these properties. Conversely, dSPN intrinsic excitability was elevated in tissue from PD models and suppressed in LID models. Although the synaptic connectivity of dSPNs did not change in PD models, it fell with L-DOPA treatment. In neither case, however, was the strength of corticostriatal connections globally scaled. Thus, SPNs manifested homeostatic adaptations in intrinsic excitability and in the number but not strength of excitatory corticostriatal synapses. The striatum is a major component of the basal ganglia circuitry controlling goal-directed action selection and habits [1] . Spiny projection neurons (SPNs) constitute the vast majority of striatal neurons and are organized into two distinct GABAergic projection systems: direct pathway SPNs (dSPNs) that directly project to the interface of the basal ganglia with the rest of the brain, promoting action selection, and indirect pathway SPNs (iSPNs) that indirectly project to the interface through the globus pallidus externa, suppressing actions [2] . These two types of SPNs are differentially modulated by dopamine released by substantia nigra pars compacta (SNc) neurons. Dopamine decreases the excitability of iSPNs through D 2 dopamine receptor (D 2 R) signalling and increases the excitability of dSPNs through D 1 dopamine receptor (D 1 R) signalling. This is accomplished through modulation of both intrinsic conductances and synaptic plasticity. Thus, event-driven changes in the spiking of SNc dopaminergic neurons bidirectionally modulate intrinsic excitability and ongoing spiking in these two SPN populations, as well as the induction of plasticity at corticostriatal synapses, shaping future SPN activity and goal-directed behaviour [3] , [4] . In Parkinson’s disease (PD), SNc dopaminergic neurons are progressively lost, disrupting this bidirectional modulation [5] , [6] . The slowness of movement and rigidity that characterize PD are attributable to hyperactivity in iSPNs and concomitant hypoactivity in dSPNs. This imbalance has long been thought to underlie the persistent action suppression characteristic of PD [7] . The administration of L-3,4-dihydroxyphenylalanine (L-DOPA)—a dopamine precursor—boosts the production and release of dopamine in the striatum, restoring basal striatal tone, the balance between direct and indirect pathways, and movement control. However, as the disease progresses and more SNc dopaminergic neurons are lost, the dose of L-DOPA needed to restore movement rises and the mechanisms for controlling extracellular dopamine are lost [8] , [9] , [10] , [11] . This combination leads to slow, poorly regulated fluctuations in extracellular dopamine concentrations. These fluctuations result in abnormally prolonged periods of D 1 R stimulation and the emergence of abnormal movements called dyskinesia [8] , [12] , [13] . Although there are a variety of striatal biochemical changes that accompany PD and L-DOPA-induced dyskinesia (LID), the synaptic and intrinsic adaptations in SPNs driven by aberrant network activity in these states are not well understood. In particular, it is not known whether homeostatic plasticity ameliorates the perturbations in spiking expected to accompany the loss and restoration of dopamine signalling. In other neurons, two types of homeostatic plasticity have been described: intrinsic and synaptic [14] . Intrinsic homeostatic plasticity refers to alterations in the postsynaptic transformation of synaptic currents into spiking; increasing or decreasing the gain of this relationship can be used to keep average spike rate within a desired range. Synaptic homeostatic plasticity refers to global alterations in the strength of synaptic connections to achieve the same endpoint. To preserve the relative importance of synaptic inputs in driving activity, synaptic strength is typically scaled; that is, all inputs are increased or decreased in strength by the same factor [15] . If cellular learning is encoded in relative synaptic weight, then scaling will preserve it. By virtue of their complementary modulation by dopamine, dSPNs and iSPNs would be expected to undergo opposite homeostatic adaptations in PD. This inference is consistent with the demonstration that following dopamine depleting lesions, iSPNs undergo a pronounced pruning of excitatory axospinous synapses, but dSPN synaptic density remains unchanged [16] . However, the changes associated with LID are more difficult to predict because of inferred alterations in dopamine receptor signalling [17] , [18] . For example, biochemical studies show that the induction of LID is accompanied by upregulation in ERK/AP-1-dependent signalling specifically in dSPNs [8] , [12] , [13] , [19] . Recent anatomical studies suggest that the lost iSPN synaptic connections are at least partially restored following high-dose L-DOPA treatment [20] , [21] , [22] . However, it is not clear from these studies whether there are intrinsic changes that accompany the alterations in synaptic connectivity or whether synaptic strength is scaled in a way that will preserve learned associations presumably stored in the strength of corticostriatal synapses. The studies reported here were designed to answer some of these questions. They show that iSPNs and dSPNs undergo largely complementary forms of intrinsic and synaptic plasticity following lesioning of SNc dopaminergic neurons and L-DOPA treatment. Many of these homeostatic changes were cell specific (that is, iSPNs decreased excitability, compensating for a loss of inhibitory D 2 R stimulation, whereas dSPNs increased excitability to compensate for a loss of excitatory D 1 R stimulation); thus, these adaptations would serve to normalize the average spiking rate of SPNs in the face of changing dopamine concentrations. However, the strength of SPN corticostriatal synapses was not globally scaled in parallel, potentially leading to alterations in the temporal pattern of activity in vivo . SPN intrinsic excitability was altered in PD and LID models One of the most prominent differences between iSPNs and dSPNs in healthy mice is their intrinsic excitability [23] , [24] , [25] . To determine whether dopamine depletion or L-DOPA treatment altered this relationship, two sets of experiments were performed to characterize somatic and dendritic excitability. The excitability of the somatic membrane and axon initial segment (AIS) was assessed by injecting current steps of increasing amplitude through the patch electrode and measuring the resultant spiking. In control iSPNs, the relationship between injected current and spike frequency was similar to that described in previous studies [26] . In iSPNs from parkinsonian mice, intrinsic excitability was depressed, as predicted by a homeostatic response to the loss of inhibitory D 2 R signalling ( Fig. 1a,b ); that is, more current was required to achieve a similar level of spiking (for example, the number of action potentials generated by 0.2 nA current injection dropped from a median of 8 in control mice to a median of 2 in parkinsonian mice ( Fig. 1a,b )). High-dose L-DOPA treatment normalized intrinsic excitability, shifting the relationship between current and spiking back into the normal range ( Fig. 1a,b ). 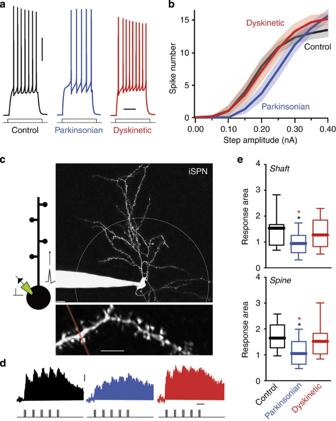Figure 1: iSPN intrinsic and dendritic excitability was reduced in iSPNs from parkinsonian mice and restored by high-dose L-DOPA. Intrinsic excitability was assessed by somatic current injection. (a) Sample traces are provided with vertical and horizontal scale bars denoting 25 mV and 200 ms, and (b) current–response curves (shaded regions illustrate s.e.m.). Intrinsic excitability was decreased in iSPNs from parkinsonian mice and restored by high-dose L-DOPA (controln=13; parkinsoniann=13; dyskineticn=12; two-way analysis of variance). Dendritic excitability was assessed by somatically driven theta burst stimulation. (c) Cartoon (left) and iSPN 2PLSM image provided (top right) with a high-magnification 2PLSM image depicting dendritic segment with a line representing the region assessed for Ca2+fluorescence (bottom); scale bars, 10 μm with an eccentricity denoting 80 μm from the soma in the low-magnification image. (d) Sample fluorescent traces provided with vertical and horizontal scale bars denoting 0.5 ΔF/F0and 200 ms, respectively. (e) Dendritic excitability was decreased in shaft (top; control median: 1.54n=17; parkinsonian median: 1.25n=19; dsykinetic median: 1.28n=24) and spine heads (bottom; control median: 1.27n=14; parkinsonian median: 1.05n=23; dyskinetic median: 1.04n=26) of parkinsonian mice and restored by high-dose L-DOPA; Kruskal–Wallis test. Sample traces provided below 2PLSM images; *P<0.05; response areas refer to (S*ΔF/F0). Other intrinsic properties of iSPNs were modestly, but often significantly changed ( Supplementary Table 1 ). For example, the amplitude of spike after-hyperpolarization was increased in iSPNs from parkinsonian mice, probably contributing to the diminished somatic/AIS excitability. Figure 1: iSPN intrinsic and dendritic excitability was reduced in iSPNs from parkinsonian mice and restored by high-dose L-DOPA. Intrinsic excitability was assessed by somatic current injection. ( a ) Sample traces are provided with vertical and horizontal scale bars denoting 25 mV and 200 ms, and ( b ) current–response curves (shaded regions illustrate s.e.m.). Intrinsic excitability was decreased in iSPNs from parkinsonian mice and restored by high-dose L-DOPA (control n =13; parkinsonian n =13; dyskinetic n =12; two-way analysis of variance). Dendritic excitability was assessed by somatically driven theta burst stimulation. ( c ) Cartoon (left) and iSPN 2PLSM image provided (top right) with a high-magnification 2PLSM image depicting dendritic segment with a line representing the region assessed for Ca 2+ fluorescence (bottom); scale bars, 10 μm with an eccentricity denoting 80 μm from the soma in the low-magnification image. ( d ) Sample fluorescent traces provided with vertical and horizontal scale bars denoting 0.5 Δ F / F 0 and 200 ms, respectively. ( e ) Dendritic excitability was decreased in shaft (top; control median: 1.54 n =17; parkinsonian median: 1.25 n =19; dsykinetic median: 1.28 n =24) and spine heads (bottom; control median: 1.27 n =14; parkinsonian median: 1.05 n =23; dyskinetic median: 1.04 n =26) of parkinsonian mice and restored by high-dose L-DOPA; Kruskal–Wallis test. Sample traces provided below 2PLSM images; * P <0.05; response areas refer to (S*Δ F / F 0 ). Full size image Although dendritic excitability in SPNs cannot be directly assessed, dendritic Ca 2+ entry evoked by back-propagating action potentials provides a surrogate measure [25] , [27] . Using two-photon laser scanning microscopy (2PLSM) to measure changes in the fluorescence of the Ca 2+ indicator Fluo-4, reliable dendritic Ca 2+ signals were evoked by theta-burst stimulation of the somatic membrane. In iSPNs from parkinsonian mice, this Ca 2+ signal was significantly reduced in distal dendritic shafts and spines ( Fig. 1c–e ). L-DOPA treatment restored iSPN dendritic excitability ( Fig. 1c–e ) (low-dose L-DOPA was also effective; shaft median: 1.4, lower quartile: 0.9, upper quartile: 1.8; head median: 1.4, lower quartile: 1.0, upper quartile: 1.9; n =16). The intrinsic excitability of dSPNs also was altered in a manner consistent with a homeostatic mechanism. In control dSPNs, the relationship between injected current and spike frequency was similar to that described in previous studies [23] . In dSPNs from parkinsonian mice, intrinsic excitability was significantly elevated, consistent with a homeostatic response to the loss of facilitating D 1 R signalling ( Fig. 2a,b ); that is, less current was required to achieve a similar level of spiking (for example, 0.2 nA current injection evoked a median of 0 spikes in control dSPNs, which increased to a median of 11 spikes in parkinsonian dSPNs; P <0.05). High-dose L-DOPA treatment partially normalized intrinsic excitability, shifting the relationship between current and spiking back towards the normal range ( Fig. 2a,b ). 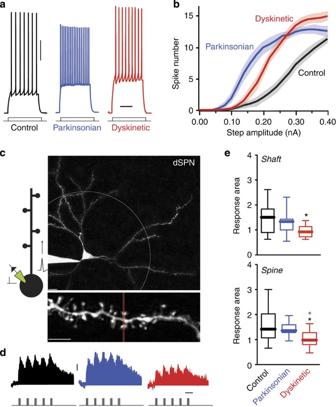Figure 2: dSPN intrinsic excitability was increased in parkinsonian mice and partially restored by high-dose L-DOPA with a decrease in dendritic excitability. (a) Sample traces are provided with vertical and horizontal scale bars denoting 25 mV and 200 ms, and (b) current–response curves (shaded regions illustrate s.e.m.). Intrinsic excitability was increased in dSPNs from parkinsonian mice and partially restored by high-dose L-DOPA (controln=24; parkinsoniann=20; dyskineticn=21; two-way analysis of variance). Dendritic excitability was assessed by somatically driven theta burst stimulation. (c) Cartoon (left) and iSPN 2PLSM image provided (top right) with a high-magnification 2PLSM image depicting dendritic segment with a line representing the region assessed for Ca2+fluorescence (bottom); scale bars, 10 μm with an eccentricity denoting 80 μm from the soma in the low-magnification image. (d) Sample fluorescent traces provided with vertical and horizontal scale bars denoting 0.5 ΔF/F0and 200 ms, respectively. (e) dSPN dendritic excitability was decreased in the dendritic shaft (top; control median: 1.52n=26; parkinsonian median: 1.01n=22; dsykinetic median: 0.94n=16) and spine heads (bottom; control median: 1.06n=21; parkinsonian median: 1.35n=24; dyskinetic median: 0.98n=17) of high-dose L-DOPA-treated mice; Kruskal–Wallis test. Sample traces provided below 2PLSM images; *P<0.05; response areas refer to (S*ΔF/F0). Other intrinsic properties of dSPNs were altered by lesioning and L-DOPA treatment ( Supplementary Table 2 ). Rheobase and action potential amplitude were decreased, whereas input resistance was increased in parkinsonian and dyskinetic mice compared with that in control. In contrast, the after-hyperpolarization amplitude was increased in dyskinetic mice compared with that in both control and parkinsonian mice, contributing to the partial restoration of soma/AIS excitability. Figure 2: dSPN intrinsic excitability was increased in parkinsonian mice and partially restored by high-dose L-DOPA with a decrease in dendritic excitability. ( a ) Sample traces are provided with vertical and horizontal scale bars denoting 25 mV and 200 ms, and ( b ) current–response curves (shaded regions illustrate s.e.m.). Intrinsic excitability was increased in dSPNs from parkinsonian mice and partially restored by high-dose L-DOPA (control n =24; parkinsonian n =20; dyskinetic n =21; two-way analysis of variance). Dendritic excitability was assessed by somatically driven theta burst stimulation. ( c ) Cartoon (left) and iSPN 2PLSM image provided (top right) with a high-magnification 2PLSM image depicting dendritic segment with a line representing the region assessed for Ca 2+ fluorescence (bottom); scale bars, 10 μm with an eccentricity denoting 80 μm from the soma in the low-magnification image. ( d ) Sample fluorescent traces provided with vertical and horizontal scale bars denoting 0.5 Δ F / F 0 and 200 ms, respectively. ( e ) dSPN dendritic excitability was decreased in the dendritic shaft (top; control median: 1.52 n =26; parkinsonian median: 1.01 n =22; dsykinetic median: 0.94 n =16) and spine heads (bottom; control median: 1.06 n =21; parkinsonian median: 1.35 n =24; dyskinetic median: 0.98 n =17) of high-dose L-DOPA-treated mice; Kruskal–Wallis test. Sample traces provided below 2PLSM images; * P <0.05; response areas refer to (S*Δ F / F 0 ). Full size image Dendritic excitability in dSPNs—as estimated by dendritic Ca 2+ signal evoked by back-propagating action potentials—was stable after 6-hydroxydopamine (6-OHDA) lesioning ( Fig. 2e ). However, after L-DOPA treatment (including low-dose L-DOPA; shaft median: 1.0, lower quartile: 0.7, upper quartile: 1.6; head median: 1.0, lower quartile: 0.8, upper quartile: 1.5; n =40), the excitability of distal dendrites fell significantly ( Fig. 2e ), in parallel with somatic excitability. Dendritic length was reduced in PD models As the difference in intrinsic excitability of dSPNs and iSPNs is partially attributable to dSPNs having larger dendritic trees than iSPNs, it is possible that the excitability changes induced by lesioning and L-DOPA treatment were a reflection of changing anatomy [23] . To test this hypothesis, the dendritic trees of iSPNs were filled with Alexa 568 and reconstructed using 2PLSM. Contrary to the predictions of this hypothesis, lesioning dopaminergic neurons significantly reduced the complexity of the iSPN dendritic arbor ( Fig. 3 ). The number of branch points as a function of distance from the soma was decreased both proximally and distally ( Fig. 3b ). Total dendritic length ( Fig. 3c ) and number of primary dendrites ( Fig. 3e ) were significantly decreased as well. Moreover, high-dose L-DOPA treatment to parkinsonian mice did not reverse the reduction iSPN dendritic branching ( Fig. 3b–e ). 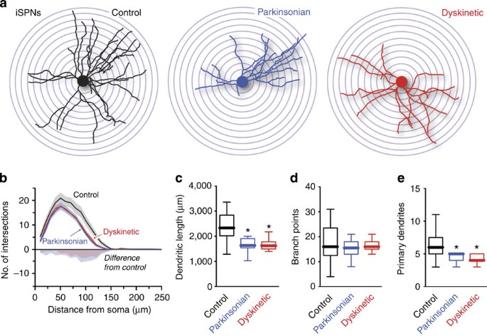Figure 3: iSPN dendritic arborization is reduced in parkinsonian mice and is not restored by high-dose L-DOPA. iSPN neurons were patched and filled with Alexa 568, 2PLSM images obtained and reconstructed in three dimensional images. (a) Representative reconstructions of iSPNs from control (black), parkinsonian (blue) and dyskinetic (red) mice with eccentricities every 10 μm from the soma. (b) Sholl analysis of reconstructed iSPNs; solid lines represent the mean with shaded regions illustrating s.e.m. (c) Total dendritic length was reduced in both parkinsonian (median: 1,627 μm) and dyskinetic mice (median: 1,622 μm) compared with that in control (median: 2,333 μm). (d) Number of branch points was unchanged by treatment conditions (control median: 12.5, parkinsonian median: 13.0, dyskinetic median: 16.0). (e) Number of primary dendrites was reduced in both parkinsonian (median: 5.0) and dyskinetic (median: 4.0) mice (control median: 6.0). Controln=14, parkinsoniann=11 and dyskineticn=12; *P<0.05; Kruskal–Wallis test. Figure 3: iSPN dendritic arborization is reduced in parkinsonian mice and is not restored by high-dose L-DOPA. iSPN neurons were patched and filled with Alexa 568, 2PLSM images obtained and reconstructed in three dimensional images. ( a ) Representative reconstructions of iSPNs from control (black), parkinsonian (blue) and dyskinetic (red) mice with eccentricities every 10 μm from the soma. ( b ) Sholl analysis of reconstructed iSPNs; solid lines represent the mean with shaded regions illustrating s.e.m. ( c ) Total dendritic length was reduced in both parkinsonian (median: 1,627 μm) and dyskinetic mice (median: 1,622 μm) compared with that in control (median: 2,333 μm). ( d ) Number of branch points was unchanged by treatment conditions (control median: 12.5, parkinsonian median: 13.0, dyskinetic median: 16.0). ( e ) Number of primary dendrites was reduced in both parkinsonian (median: 5.0) and dyskinetic (median: 4.0) mice (control median: 6.0). Control n =14, parkinsonian n =11 and dyskinetic n =12; * P <0.05; Kruskal–Wallis test. Full size image As with iSPNs, lesioning dopaminergic neurons significantly reduced the complexity of the dSPN dendritic arbor ( Fig. 4a ). The number of branch points as a function of distance from the soma was decreased both proximally and distally ( Fig. 4b ). Total dendritic length, number of branch points and number of primary dendrites were significantly decreased ( Fig. 4c–e ). Dyskinesiogneic L-DOPA treatment to parkinsonian mice did not reverse the reduction dSPN dendritic branching. Extending L-DOPA treatment for 28 days (injections every other day) did not restore dendrites either ( Supplementary Fig. 2 ). 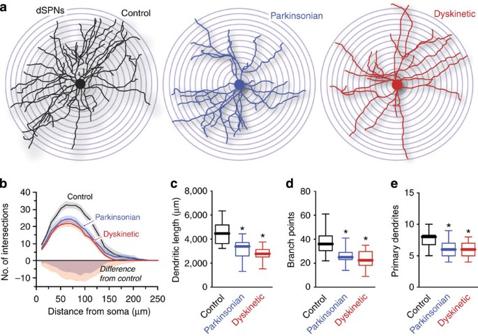Figure 4: dSPN dendritic arborization is reduced in parkinsonian mice and is not restored by high-dose L-DOPA. dSPN neurons were patched and filled with Alexa 568, 2PLSM images obtained and reconstructed in three-dimensional images. (a) Representative reconstructions of iSPNs from control (black), parkinsonian (blue) and dyskinetic (red) mice with eccentricities every 10 μm from the soma. (b) Sholl analysis of reconstructed dSPNs; solid lines represent the mean with shaded regions illustrating s.e.m. (c) Total dendritic length was reduced in parkinsonian (median: 3,388 μm) and dyskinetic mice (median: 2,774 μm) compared with control (median: 4,464 μm). (d) Number of branch points was decreased in both parkinsonian (median: 25) and dyskinetic (median: 22.5) mice compared with control (median: 36). (e) Number of primary dendrites was decreased in parkinsonian (median: 6) and dyskinetic mice (median: 6) compared with control (median: 8). Controln=13, parkinsoniann=13 and dyskineticn=11; *P<0.05; Kruskal–Wallis test. Figure 4: dSPN dendritic arborization is reduced in parkinsonian mice and is not restored by high-dose L-DOPA. dSPN neurons were patched and filled with Alexa 568, 2PLSM images obtained and reconstructed in three-dimensional images. ( a ) Representative reconstructions of iSPNs from control (black), parkinsonian (blue) and dyskinetic (red) mice with eccentricities every 10 μm from the soma. ( b ) Sholl analysis of reconstructed dSPNs; solid lines represent the mean with shaded regions illustrating s.e.m. ( c ) Total dendritic length was reduced in parkinsonian (median: 3,388 μm) and dyskinetic mice (median: 2,774 μm) compared with control (median: 4,464 μm). ( d ) Number of branch points was decreased in both parkinsonian (median: 25) and dyskinetic (median: 22.5) mice compared with control (median: 36). ( e ) Number of primary dendrites was decreased in parkinsonian (median: 6) and dyskinetic mice (median: 6) compared with control (median: 8). Control n =13, parkinsonian n =13 and dyskinetic n =11; * P <0.05; Kruskal–Wallis test. Full size image These results suggest that the intrinsic homeostatic plasticity seen in response to lesioning and L-DOPA treatment were not attributable to changes in dendritic anatomy. Furthermore, as these changes were qualitatively similar in dSPNs and iSPNs, and unaltered by L-DOPA treatment, it is likely to be that the dendrites were responding to some factor other than dopamine that was lost by lesioning mesencephalic neurons. L-DOPA treatment altered spine density As previously described [16] , lesioning of the dopaminergic innervation was accompanied by a significant reduction in iSPN spine density ( Fig. 5 ). The reduction was found in both proximal (<80 μm from the soma) and distal (>80 μm from the soma) dendrites. High-dose L-DOPA treatment, but not low-dose L-DOPA (proximal median: 0.7, lower quartile: 0.5, upper quartile: 0.9; distal median: 0.7, lower quartile: 0.6, upper quartile: 0.8; n =9), reversed this loss, bringing spine density in both proximal and distal dendrites to values that were not significantly different from controls ( Fig. 5 ). Despite the restoration in spine density with high-dose L-DOPA, estimates of total spine number remained below control levels as a result of decreased dendritic length ( Fig. 5e ). 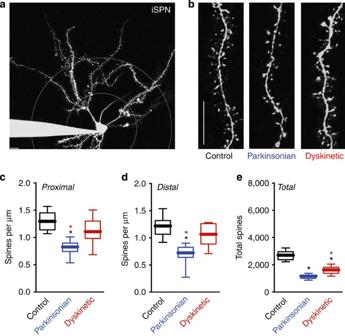Figure 5: iSPN axospinous synapses were reduced in parkinsonian mice and restored by high-dose L-DOPA. (a) 2PLSM image of an iSPN (left) from a control mouse with circles delineating minimal proximal (40 μm) and distal (80 μm) distances from the soma. (b) Representative 2PLSM images of proximal dendritic segments from control (black), parkinsonian (blue) and dyskinetic (red) mice. (c) iSPN proximal spine density was decreased in parkinsonian mice (median: 0.83 spines per μm) and restored in dyskinetic mice (median: 1.11 spines per μm; control median: 1.30 spines per μm). (d) iSPN distal spine density was also decreased in parkinsonian mice (median: 0.64 spines perμm) and restored in dyskinetic mice (median 1.07 spines per μm; control median: 1.22 spines per μm). (e) Total number of spines were estimated based on spine density and dendritic anatomy data (Fig. 3); despite a restoration in spine density with dyskinesia, total number of spines remain below control levels due to reduced dendritic surface area. Total spine estimates for control median: 2,701 spines, parkinsonian median: 1,171 spines and dyskinetic median: 1,622 spines; controln=16, parkinsoniann=17, dyskineticn=15; *P<0.05; scale bar, 10 μm; Kruskal–Wallis test. Figure 5: iSPN axospinous synapses were reduced in parkinsonian mice and restored by high-dose L-DOPA. ( a ) 2PLSM image of an iSPN (left) from a control mouse with circles delineating minimal proximal (40 μm) and distal (80 μm) distances from the soma. ( b ) Representative 2PLSM images of proximal dendritic segments from control (black), parkinsonian (blue) and dyskinetic (red) mice. ( c ) iSPN proximal spine density was decreased in parkinsonian mice (median: 0.83 spines per μm) and restored in dyskinetic mice (median: 1.11 spines per μm; control median: 1.30 spines per μm). ( d ) iSPN distal spine density was also decreased in parkinsonian mice (median: 0.64 spines perμm) and restored in dyskinetic mice (median 1.07 spines per μm; control median: 1.22 spines per μm). ( e ) Total number of spines were estimated based on spine density and dendritic anatomy data ( Fig. 3 ); despite a restoration in spine density with dyskinesia, total number of spines remain below control levels due to reduced dendritic surface area. Total spine estimates for control median: 2,701 spines, parkinsonian median: 1,171 spines and dyskinetic median: 1,622 spines; control n =16, parkinsonian n =17, dyskinetic n =15; * P <0.05; scale bar, 10 μm; Kruskal–Wallis test. Full size image In agreement with previous work [16] , dSPN spine density did not change significantly following 6-OHDA lesioning ( Fig. 6 ). However, because of the loss of dendritic length, the estimated total number of dSPN axospinous synapses fell with lesioning. In contrast, both proximal and distal spine density in dSPNs fell with low-dose L-DOPA (proximal median: 0.8, lower quartile: 0.7, upper quartile: 1.1 n =10; distal median: 0.8, lower quartile: 0.6, upper quartile: 0.8; n =13) and high-dose L-DOPA treatment ( Fig. 6c,d ), as did the estimate of total number of spines ( Fig. 6e ). 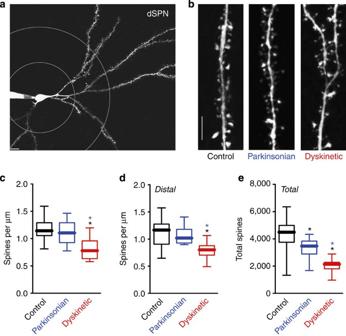Figure 6: dSPN axospinous synapses were reduced in L-DOPA-treated mice. (a) 2PLSM image of a dSPN (left) from a control mouse with circles delineating minimal proximal (40 μm) and distal (80 μm) distances from the soma. (b) Representative 2PLSM images of proximal dendritic segments from control, parkinsonian and dyskinetic mice. dSPN proximal (c) and distal (d) spine density was decreased in L-DOPA-treated mice compared with controls. (e) Total number of spines were estimated based on spine density and dendritic anatomy data (Fig. 4); dyskinetic mice (median: 2,096) had fewer spines than control (median: 4,715) and parkinsonian mice (median: 3,426); controln=16, parkinsoniann=17, dyskineticn=15; *P<0.05; scale bar, 10 μm; Kruskal–Wallis test. Figure 6: dSPN axospinous synapses were reduced in L-DOPA-treated mice. ( a ) 2PLSM image of a dSPN (left) from a control mouse with circles delineating minimal proximal (40 μm) and distal (80 μm) distances from the soma. ( b ) Representative 2PLSM images of proximal dendritic segments from control, parkinsonian and dyskinetic mice. dSPN proximal ( c ) and distal ( d ) spine density was decreased in L-DOPA-treated mice compared with controls. ( e ) Total number of spines were estimated based on spine density and dendritic anatomy data ( Fig. 4 ); dyskinetic mice (median: 2,096) had fewer spines than control (median: 4,715) and parkinsonian mice (median: 3,426); control n =16, parkinsonian n =17, dyskinetic n =15; * P <0.05; scale bar, 10 μm; Kruskal–Wallis test. Full size image Adaptations in corticostriatal connectivity To determine the functional significance of changes in spine density ( Figs 5 and 6 ), electrophysiological and/or optogenetic studies were conducted. As a first step, the source of the presynaptic element at axospinous synapses was determined. In control rodents, the vast majority of these axospinous synapses are corticostriatal [28] , [29] . To interrogate corticostriatal axospinous circuitry, Thy1-ChR2 transgenic mice were used [30] . In these mice, channelrhodopsin (ChR2) expression in glutamatergic neurons appears to be limited to corticostriatal pyramidal neurons and not extend to thalamostriatal neurons [31] . To map corticostriatal synapses, the sCRACm approach [32] was used in ex vivo brain slices from bitransgenic mice expressing ChR2 in cortical neurons and a fluorescent reporter of SPN subtype [31] . At spines where there was a cortical terminal expressing ChR2, a blue laser flash induced glutamate release, which was detected as a postsynaptic current ( Figs 7 and 8 ). 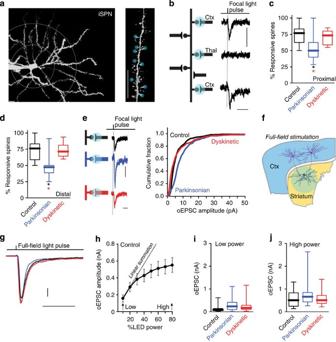Figure 7: Cortical axospinous synapses in iSPNs were lost in parkinsonian mice and rewired with high-dose L-DOPA. sCRACm was used to assess corticostriatal circuit function in iSPNs from control (black), parkinsonian (blue) and dyskinetic (red) mice. (a) Sample 2PLSM image depicting a patched iSPN (left) and dendritic region (right) assessed for functional corticostriatal circuitry; scale bars, 10 μm. Blue circles depict region stimulated by focal blue laser excitation of ChR2. (b) The cartoon segment of dendrite shows both cortical and thalamic input onto spines and shaft. Only axospinous synapses were tested for cortical circuitry; to the right of the experimental depiction are sample traces showing responses from a corticostriatal synapse, a presumed thalamostriatal synapse and a second corticostriatal synapse; scale bar, 5 pA (vertical) and 50 ms (horizontal). Both proximal (c) and distal (d) corticostriatal axospinous synapses were lost in iSPNs from parkinsonian mice and restored by dykinesiogenic L-DOPA (proximal medians: control 76.92%n=15, parkinsonian 50.00%n=15, dyskinetic 73.33%,n=15; distal medians: control 76.19%n=15, parkinsonian 47.37%n=13, dyskinetic 71.43%,n=15). (e) Individual corticostriatal optogenetically evoked EPSCs (oEPSC) were measured, representative traces are shown to the right of experimental diagram; scale bar, 5 pA (vertical) and 50 ms (horizontal). oEPSC amplitude was increased in iSPNs from parkinsonian mice and restored in dyskinetic mice. Full-field stimulation using a blue LED was used to assess overall circuit strength. (f) Overall circuit strength was unchanged despite losing axospinous synapses parkinsonian mice sample traces provided (g) with vertical scale and horizontal scale bars denoting 100 pA and 100 ms, respectively. (h) Input–output curve demonstrating sublinearity of recorded data (solid line) and estimated linear summation (dashed line) from control cells. Box and whisker plots of minimal LED stimulation (i) (control median: 86.67 pAn=15, parkinsonian median: 237.7 pAn=15, dyskinetic median: 170.3 pAn=15) and maximal stimulation (j) (control median: 508.0 pAn=15, parkinsonian median: 660.6 pAn=15, dyskinetic median: 508.4 pAn=15) demonstrate the lack of change in overall corticostriatal circuit strength. *P<0.05; Kruskal–Wallis test. Figure 7: Cortical axospinous synapses in iSPNs were lost in parkinsonian mice and rewired with high-dose L-DOPA. sCRACm was used to assess corticostriatal circuit function in iSPNs from control (black), parkinsonian (blue) and dyskinetic (red) mice. ( a ) Sample 2PLSM image depicting a patched iSPN (left) and dendritic region (right) assessed for functional corticostriatal circuitry; scale bars, 10 μm. Blue circles depict region stimulated by focal blue laser excitation of ChR2. ( b ) The cartoon segment of dendrite shows both cortical and thalamic input onto spines and shaft. Only axospinous synapses were tested for cortical circuitry; to the right of the experimental depiction are sample traces showing responses from a corticostriatal synapse, a presumed thalamostriatal synapse and a second corticostriatal synapse; scale bar, 5 pA (vertical) and 50 ms (horizontal). Both proximal ( c ) and distal ( d ) corticostriatal axospinous synapses were lost in iSPNs from parkinsonian mice and restored by dykinesiogenic L-DOPA (proximal medians: control 76.92% n =15, parkinsonian 50.00% n =15, dyskinetic 73.33%, n =15; distal medians: control 76.19% n =15, parkinsonian 47.37% n =13, dyskinetic 71.43%, n =15). ( e ) Individual corticostriatal optogenetically evoked EPSCs (oEPSC) were measured, representative traces are shown to the right of experimental diagram; scale bar, 5 pA (vertical) and 50 ms (horizontal). oEPSC amplitude was increased in iSPNs from parkinsonian mice and restored in dyskinetic mice. Full-field stimulation using a blue LED was used to assess overall circuit strength. ( f ) Overall circuit strength was unchanged despite losing axospinous synapses parkinsonian mice sample traces provided ( g ) with vertical scale and horizontal scale bars denoting 100 pA and 100 ms, respectively. ( h ) Input–output curve demonstrating sublinearity of recorded data (solid line) and estimated linear summation (dashed line) from control cells. Box and whisker plots of minimal LED stimulation ( i ) (control median: 86.67 pA n =15, parkinsonian median: 237.7 pA n =15, dyskinetic median: 170.3 pA n =15) and maximal stimulation ( j ) (control median: 508.0 pA n =15, parkinsonian median: 660.6 pA n =15, dyskinetic median: 508.4 pA n =15) demonstrate the lack of change in overall corticostriatal circuit strength. * P <0.05; Kruskal–Wallis test. 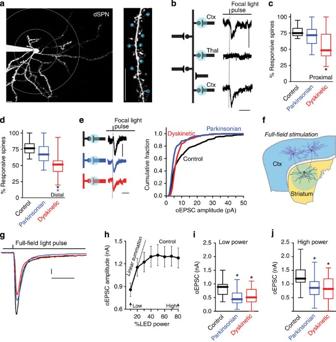Figure 8: Cortical axospinous synapses in dSPNs were lost in dyskinetic mice. sCRACm was used to assess corticostriatal circuit function in iSPNs from control (black), parkinsonian (blue) and dyskinetic (red) mice. (a) Sample 2PLSM image depicting a patched dSPN (left) and dendritic region (right) assessed for functional corticostriatal circuitry; scale bars, 10 μm. Blue circles depict region stimulated by focal blue laser excitation of ChR2. (b) The cartoon segment of dendrite shows both cortical and thalamic input onto spines and shaft. Only axospinous synapses were tested for cortical circuitry; to the right of the experimental depiction are sample traces showing responses from a corticostriatal synapse, a presumed thalamostriatal synapse and a second corticostriatal synapse; scale bar, 5 pA (vertical) and 50 ms (horizontal). Both proximal (c) and distal (d) corticostriatal axospinous synapses were lost in dSPNs from dyskinetic mice (proximal medians: control 75.00%n=13, parkinsonian 71.82%n=14 and dyskinetic 48.53%n=18; distal medians: control 76.47%n=13, parkinsonian 66.97%n=14 and dyskinetic 51.47%n=14). (e) Individual corticostriatal optogenetically evoked EPSCs (oEPSC) were measured, representative traces are shown to the right of experimental diagram; scale bar, 5 pA (vertical) and 50 ms (horizontal). EPSC amplitude data were separated into low and high EPSC amplitude groups by the median; in parkinsonian and dyskinetic mice, there were fewer high-amplitude synapses than in controls. Full-field stimulation using a blue LED was used to assess overall circuit strength. (f) Overall circuit strength was reduced in parkinsonian and dyskinetic mice; sample traces provided (g) with vertical scale and horizontal scale bars denoting 100 pA and 100 ms, respectively. (h) Input–output curve demonstrating sublinearity of recorded data (solid line) and estimated linear summation (dashed line) from control cells. Box and whisker plots of minimal LED stimulation (i) (control median: 885.4 pAn=13, parkinsonian median: 435.8 pAn=15 and dyskinetic median: 505.6 pAn=11) and maximal stimulation (j) (control median: 1,198.0 pAn=13, parkinsonian median: 857.8 pAn=15 and dyskinetic median: 817.5 pAn=11) demonstrate the decreased corticostriatal circuit strength in parkinsonian and dyskinetic mice. *P<0.05; Kruskal–Wallis and Mann–Whitney tests. Full size image Figure 8: Cortical axospinous synapses in dSPNs were lost in dyskinetic mice. sCRACm was used to assess corticostriatal circuit function in iSPNs from control (black), parkinsonian (blue) and dyskinetic (red) mice. ( a ) Sample 2PLSM image depicting a patched dSPN (left) and dendritic region (right) assessed for functional corticostriatal circuitry; scale bars, 10 μm. Blue circles depict region stimulated by focal blue laser excitation of ChR2. ( b ) The cartoon segment of dendrite shows both cortical and thalamic input onto spines and shaft. Only axospinous synapses were tested for cortical circuitry; to the right of the experimental depiction are sample traces showing responses from a corticostriatal synapse, a presumed thalamostriatal synapse and a second corticostriatal synapse; scale bar, 5 pA (vertical) and 50 ms (horizontal). Both proximal ( c ) and distal ( d ) corticostriatal axospinous synapses were lost in dSPNs from dyskinetic mice (proximal medians: control 75.00% n =13, parkinsonian 71.82% n =14 and dyskinetic 48.53% n =18; distal medians: control 76.47% n =13, parkinsonian 66.97% n =14 and dyskinetic 51.47% n =14). ( e ) Individual corticostriatal optogenetically evoked EPSCs (oEPSC) were measured, representative traces are shown to the right of experimental diagram; scale bar, 5 pA (vertical) and 50 ms (horizontal). EPSC amplitude data were separated into low and high EPSC amplitude groups by the median; in parkinsonian and dyskinetic mice, there were fewer high-amplitude synapses than in controls. Full-field stimulation using a blue LED was used to assess overall circuit strength. ( f ) Overall circuit strength was reduced in parkinsonian and dyskinetic mice; sample traces provided ( g ) with vertical scale and horizontal scale bars denoting 100 pA and 100 ms, respectively. ( h ) Input–output curve demonstrating sublinearity of recorded data (solid line) and estimated linear summation (dashed line) from control cells. Box and whisker plots of minimal LED stimulation ( i ) (control median: 885.4 pA n =13, parkinsonian median: 435.8 pA n =15 and dyskinetic median: 505.6 pA n =11) and maximal stimulation ( j ) (control median: 1,198.0 pA n =13, parkinsonian median: 857.8 pA n =15 and dyskinetic median: 817.5 pA n =11) demonstrate the decreased corticostriatal circuit strength in parkinsonian and dyskinetic mice. * P <0.05; Kruskal–Wallis and Mann–Whitney tests. Full size image In sham lesioned mice, ~75% of the iSPN spines responded to blue laser flashes ( Fig. 7c,d ), consistent with prior studies [31] . This was true in both proximal and distal dendrites. This percentage is very close to that predicted from anatomical studies [29] , [33] . In collateral studies where intralaminar thalamic neurons were induced to express ChR2, about 30% of iSPN spines were found to be responsive, suggesting that few, if any, spines had ‘silent’ synapses [31] . Following 6-OHDA lesioning, the percentage of spines with a detectable cortical terminal fell to ~40% ( Fig. 7c,d ). Thus, lesion-induced spine pruning was prominent at corticostriatal axospinous synapses. Surprisingly, following high-dose L-DOPA treatment, the proportion of spines responsive to optogenetic activation of corticostriatal terminals returned to near-control values ( Fig. 7c,d ). In addition to the presence of functional α-amino-3-hydroxy-5-methyl-4-isoxazolepropionic acid receptors (AMPARs), the sCRACm mapping yields information about synaptic strength. Following 6-OHDA lesioning, the average amplitude of corticostriatal synaptic responses in iSPNs increased ( Fig. 7e ), in agreement with previous work using electrical stimulation of cortical axons and Ca 2+ replacement with Sr 2+ (ref. 34 ). High-dose L-DOPA treatment normalized the amplitude of the corticostriatal responses ( Fig. 7e ). These changes are consistent with the known role of D 2 R signalling in promoting long-term depression of corticostriatal synapses [2] , [35] . However, they were not consistent with homeostatic scaling, which would predict a downward (leftward) shift in synaptic strength in the PD model and an upward (rightward) shift in the LID model. Rather, excitatory synaptic strength increased in the PD model when iSPN intrinsic excitability was falling and then decreased when iSPN intrinsic excitability was rising in the LID model. To provide an additional level of confidence that this pattern was not the product of the optogenetic approach, Sr 2+ miniature excitatory postsynaptic currents (mEPSCs) evoked by cortical stimulation in parasagittal brain slices were examined. As the parkinsonian condition had been examined previously [34] , these studies focused on the LID model. As predicted from the optogenetic experiments, corticostriatal Sr 2+ mEPSC amplitude in the sham and L-DOPA-treated conditions was not significantly different (sham median: 14.13 pA, lower quartile: 12.63 pA, upper quartile: 15.25 pA, n =8; dyskinetic median: 14.85 pA, lower quartile: 12.85 pA, upper quartile: 16.46 pA, n =10; Mann–Whitney test, P =0.49). The data shown demonstrate that following lesioning of dopamine neurons the number of corticostriatal synapses on iSPNs fell, but their average strength rose. Conversely, with high-dose L-DOPA treatment the number of corticostriatal synapses rose, but their average strength fell. The opposing alterations in number and strength of synapses might effectively cancel one another, leaving total synaptic currents constant. To test this prediction, iSPNs were loaded with Cs + to make them as electrotonically compact as possible and to lessen the impact of the changes in dendritic excitability described above; then, corticostriatal axons were optogenetically stimulated by a full-field blue light flash. In iSPNs from sham lesioned mice (as well as those from treated mice) the optogenetically evoked synaptic response was sublinearly related to stimulus intensity ( Fig. 7h ); this was expected as progressively larger dendritic depolarization diminishes the driving force for synaptic currents. Nevertheless, at both low and high stimulation intensities, the evoked synaptic responses of iSPNs in slices from control, parkinsonian and LID mice were indistinguishable ( Fig. 7i,j ). dSPN corticostriatal connectivity fell in the LID model. As with iSPNs, electrophysiological and optogenetic approaches were used to characterize the properties of dSPN synapses in each model. The origin of the presynaptic element at axospinous synapses was determined using sCRACm, as described above. In control and lesioned Thy1-ChR2 mice, ~75% of the dSPN spines responded to optogenetic activation ( Fig. 8c,d ). This was true in both proximal and distal dendrites. The percentage was indistinguishable from that in iSPNs. Following high-dose L-DOPA treatment, this percentage fell significantly ( Fig. 8c,d ), demonstrating that corticostriatal synapses were being pruned. The sCRACm approach also was used to determine whether there were alterations in synaptic strength following LID induction. In dSPNs from both parkinsonian and LID mice, there was a significant reduction in the relative abundance of large amplitude corticostriatal synaptic currents ( Fig. 8e ). However, using electrical stimulation of sensorimotor cortex axons and Sr 2+ replacement of extracellular Ca 2+ to generate asynchronous miniature EPSCs, no differences were seen in the distribution of synaptic amplitudes across conditions (control median: 15.2 pA, lower quartile: 11.5 pA, upper quartile: 17.2 pA, n =17; parkinsonian median: 14.9 pA, lower quartile: 13.5 pA, upper quartile: 17.0 pA, n =12; dyskinetic median: 14.2 pA, lower quartile: 12.7 pA, upper quartile: 15.8 pA, n =13; Kruskal–Wallis test, P =0.70). Given that many regions of cortex project to SPNs [36] , it is possible that this apparent discrepancy is a consequence of preferential downregulating synaptic connections arising from limbic or sensory cortical regions (which were not assayed in Sr 2+ experiments) following LID induction. Taken together, these results suggest that in the absence of dopamine (that is, in parkinsonian and LID mice during the ‘off-state’), there was a reduction in the total strength of corticostriatal synapses on dSPNs. This reduction in synaptic strength was complemented in the LID model by a reduction in the number of corticostriatal axospinous synapses. As a consequence, the aggregate cortical synaptic response in dSPNs should be smaller in tissue from PD and LID models. To test this prediction, the cortical inputs to dSPNs were optogenetically stimulated in the Thy1-ChR2 transgenic mice. As with iSPNs, the optogenetically evoked post-synaptic currents were sublinearly related to stimulus intensity ( Fig. 8h ). More importantly, the evoked synaptic response of dSPNs in slices from PD and LID mice was smaller than that in tissue from control mice at both low and high stimulation intensities ( Fig. 8i,j ). Extrasynaptic NMDAR currents were correlated with spine loss Another feature of striatal glutamatergic synaptic transmission that has been reported to change with lesioning of the dopaminergic neurons and LID is the balance between synaptic and extrasynaptic N -methyl- D -aspartate receptors (NMDARs) [37] . However, none of the studies that have been conducted to date have distinguished between glutamatergic synapses on iSPNs and dSPNs. To fill this gap, iSPNs were patch clamped and the ratio between NMDAR and AMPAR currents measured. Initially, the NMDAR/AMPAR ratio was assessed using two-photon laser uncaging of glutamate on spine heads. These studies revealed that the NMDAR/AMPAR at iSPN spines increased following 6-OHDA lesioning and then returned to normal values after high-dose L-DOPA treatment ( Fig. 9c ) and low-dose L-DOPA (median: 1.1, lower quartile: 0.9, upper quartile: 1.6; n =55). 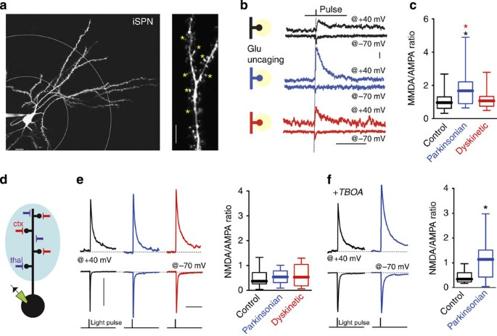Figure 9: Extrasynaptic NMDA/AMPA ratios in iSPNs were increased in parkinsonian mice. (a) 2PLSM image depicting an iSPN (left) with circles delineating proximal (40 μm from soma) and distal (80 μm from soma) dendritic segments and a high-magnification image of a dendritic segment (middle) with yellow asterisks indicating regions targeted with uncaging laser; scale bars, 10 μm. To the right is a cartoon depicting regions exposed to glutamate due to uncaging (yellow circles). (b) Sample traces depicting uncaged glutamate-induced responses used to assess NMDA/AMPA ratios (middle) and data from control (black), parkinsonian (blue) and dyskinetic mice (red); vertical and horizontal scale bars denote 10 pA and 100 ms, respectively. (c) NMDA/AMPA ratios in iSPNs were increased in parkinsonian mice (control median: 0.96n=58 spines; parkinsonian median: 1.67n=44 spines; dyskinetic median: 1.07n=43 spines). (d) Cartoon depicting full-field stimulation of an iSPN exciting all cortical inputs. (e) Synaptic NMDA/AMPA ratios (determined using cortical optogenetic stimulation) with sample traces on the left and data showing no change on the right; vertical and horizontal scale bars denote 100 pA and 100 ms, respectively (control median: 0.37n=16; parkinsonian median: 0.54n=17; dyskinetic median: 0.54n=16). (f) To verify findings with uncaged glutamate, full-field optogenetic stimulation was again tested in the presence of DL-threo-β-benzyloxyaspartic acid (TBOA) to engage both synaptic and extrasynaptic receptors. Sample traces provided on the left; again, NMDA/AMPA ratio was increased in parkinsonian mice, verifying that changes were due to extrasynaptic receptors (control median: 0.35n=13; parkinsonian median: 1.14n=16). *P<0.05; Kruskal–Wallis and Mann–Whitney tests. Figure 9: Extrasynaptic NMDA/AMPA ratios in iSPNs were increased in parkinsonian mice. ( a ) 2PLSM image depicting an iSPN (left) with circles delineating proximal (40 μm from soma) and distal (80 μm from soma) dendritic segments and a high-magnification image of a dendritic segment (middle) with yellow asterisks indicating regions targeted with uncaging laser; scale bars, 10 μm. To the right is a cartoon depicting regions exposed to glutamate due to uncaging (yellow circles). ( b ) Sample traces depicting uncaged glutamate-induced responses used to assess NMDA/AMPA ratios (middle) and data from control (black), parkinsonian (blue) and dyskinetic mice (red); vertical and horizontal scale bars denote 10 pA and 100 ms, respectively. ( c ) NMDA/AMPA ratios in iSPNs were increased in parkinsonian mice (control median: 0.96 n =58 spines; parkinsonian median: 1.67 n =44 spines; dyskinetic median: 1.07 n =43 spines). ( d ) Cartoon depicting full-field stimulation of an iSPN exciting all cortical inputs. ( e ) Synaptic NMDA/AMPA ratios (determined using cortical optogenetic stimulation) with sample traces on the left and data showing no change on the right; vertical and horizontal scale bars denote 100 pA and 100 ms, respectively (control median: 0.37 n =16; parkinsonian median: 0.54 n =17; dyskinetic median: 0.54 n =16). ( f ) To verify findings with uncaged glutamate, full-field optogenetic stimulation was again tested in the presence of DL-threo-β-benzyloxyaspartic acid (TBOA) to engage both synaptic and extrasynaptic receptors. Sample traces provided on the left; again, NMDA/AMPA ratio was increased in parkinsonian mice, verifying that changes were due to extrasynaptic receptors (control median: 0.35 n =13; parkinsonian median: 1.14 n =16). * P <0.05; Kruskal–Wallis and Mann–Whitney tests. Full size image Although these studies demonstrate an important postsynaptic adaptation, they suffer from two limitations. First, even when the intensity of the uncaging laser is adjusted to mimic naturally occurring minimal synaptic events (~5 pA), there was no certainty that only synaptic receptors are being stimulated. Second, the type of synapse (corticostriatal or thalamostriatal) was unknown. Overcoming these limitations is important for a number of reasons, not the least of which is that the NMDAR/AMPAR of thalamostriatal and corticostriatal synapses differ in control mice, making sampling bias a potential factor [38] . To address these shortcomings, corticostriatal axons were optically stimulated in slices from Thy1 transgenic mice described above and the NMDAR/AMPAR ratio measured. In normal recording conditions, this ratio did not change as a function of treatment condition ( Fig. 9e ). However, when glutamate uptake was blocked using DL-threo-β-benzyloxyaspartic acid, the NMDAR/AMPAR ratio was significantly elevated following 6-OHDA lesioning ( Fig. 9f ). These data are consistent with the proposition that the abundance of iSPN extrasynaptic NMDARs increased at corticostriatal axospinous synapses following loss of dopaminergic innervation and then returned to normal as corticostriatal synaptic density rose with LID. To determine whether these changes were common to SPNs, dSPNs were patch clamped and the ratio between NMDAR and AMPAR currents measured. Two-photon laser uncaging of glutamate on spine heads revealed that the NMDAR-to-AMPAR current ratio at dSPN spines was unchanged following 6-OHDA lesioning and then increased after L-DOPA administration ( Fig. 10c ), including low-dose L-DOPA (median: 1.4, lower quartile: 1.0, upper quartile: 2.1; n =60). To link these observations to synaptic transmission, corticostriatal axons were optically stimulated and the NMDAR-to-AMPAR current ratio measured. In normal recording conditions, this ratio did not change as a function of treatment condition ( Fig. 10e ). However, when glutamate uptake was blocked using DL-threo-β-benzyloxyaspartic acid, the NMDAR-to-AMPAR current ratio was significantly elevated in tissue from LID mice ( Fig. 10f ). These data are consistent with the proposition that the abundance of dSPN extrasynaptic NMDARs was unchanged at corticostriatal axospinous synapses following loss of dopaminergic innervation and then rose as corticostriatal synaptic density fell with high-dose L-DOPA treatment. 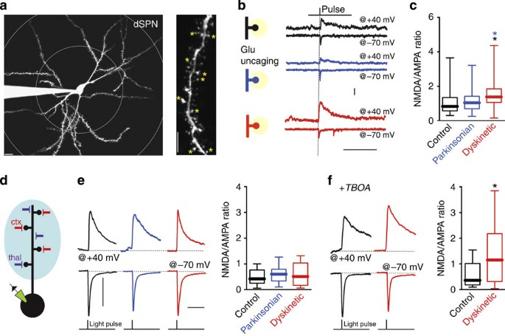Figure 10: Extrasynaptic NMDA/AMPA ratios in dSPNs were increased in dyskinetic mice. (a) 2PLSM image depicting a dSPN (left) with circles delineating proximal (40 μm from soma) and distal (80 μm from soma) dendritic segments, and a high-magnification image of a dendritic segment (middle) with yellow asterisks indicating regions targeted with uncaging laser; scale bars, 10 μm. To the right is a cartoon depicting regions exposed to glutamate due to uncaging (yellow circles). (b) Sample traces depicting uncaged glutamate-induced responses used to assess NMDA/AMPA ratios (middle) and data from control (black), parkinsonian (blue) and dyskinetic mice (red); vertical and horizontal scale bars denote 10 pA and 100 ms, respectively. (c) NMDA/AMPA ratios in dSPNs were increased in dyskinetic mice (control median: 0.81n=61 spines; parkinsonian median: 0.58n=46 spines; dyskinetic median: 1.04n=55 spines). (d) Cartoon depicting full-field stimulation with a dSPN exciting all cortical inputs. (e) Synaptic NMDA/AMPA ratios (determined using cortical optogenetic stimulation) with sample traces on the left and data showing no change on the right; vertical and horizontal scale bars denote 100 pA and 100 ms, respectively (control median: 0.43n=13; parkinsonian median: 0.61n=13; dyskinetic median: 0.52n=14). (f) To verify findings with uncaged glutamate, full-field optogenetic stimulation was again tested in the presence of DL-threo-β-benzyloxyaspartic acid (TBOA) to engage both synaptic and extrasynaptic receptors. Sample traces provided on the left; again, NMDA/AMPA ratio was increased in parkinsonian mice, verifying that changes were due to extrasynaptic receptors (control median: 0.37n=17; parkinsonian median: 1.16n=15). *P<0.05; Kruskal–Wallis and Mann–Whitney tests. Figure 10: Extrasynaptic NMDA/AMPA ratios in dSPNs were increased in dyskinetic mice. ( a ) 2PLSM image depicting a dSPN (left) with circles delineating proximal (40 μm from soma) and distal (80 μm from soma) dendritic segments, and a high-magnification image of a dendritic segment (middle) with yellow asterisks indicating regions targeted with uncaging laser; scale bars, 10 μm. To the right is a cartoon depicting regions exposed to glutamate due to uncaging (yellow circles). ( b ) Sample traces depicting uncaged glutamate-induced responses used to assess NMDA/AMPA ratios (middle) and data from control (black), parkinsonian (blue) and dyskinetic mice (red); vertical and horizontal scale bars denote 10 pA and 100 ms, respectively. ( c ) NMDA/AMPA ratios in dSPNs were increased in dyskinetic mice (control median: 0.81 n =61 spines; parkinsonian median: 0.58 n =46 spines; dyskinetic median: 1.04 n =55 spines). ( d ) Cartoon depicting full-field stimulation with a dSPN exciting all cortical inputs. ( e ) Synaptic NMDA/AMPA ratios (determined using cortical optogenetic stimulation) with sample traces on the left and data showing no change on the right; vertical and horizontal scale bars denote 100 pA and 100 ms, respectively (control median: 0.43 n =13; parkinsonian median: 0.61 n =13; dyskinetic median: 0.52 n =14). ( f ) To verify findings with uncaged glutamate, full-field optogenetic stimulation was again tested in the presence of DL-threo-β-benzyloxyaspartic acid (TBOA) to engage both synaptic and extrasynaptic receptors. Sample traces provided on the left; again, NMDA/AMPA ratio was increased in parkinsonian mice, verifying that changes were due to extrasynaptic receptors (control median: 0.37 n =17; parkinsonian median: 1.16 n =15). * P <0.05; Kruskal–Wallis and Mann–Whitney tests. Full size image A summary of the collective findings are provided in Supplementary Table 3 . There are four general conclusions that can be drawn from our studies. First, the loss of dopaminergic neurons innervating the striatum induces dendritic atrophy in both dSPNs and iSPNs through a mechanism that appears to be independent of dopamine. Second, both iSPNs and dSPNs manifest intrinsic and synaptic forms of homeostatic plasticity that should mitigate perturbations in average spiking rate accompanying PD and LID states. Third, global synaptic scaling was not a feature of the SPN adaptations in either PD or LID models. Fourth, the only adaptation found to be exclusively associated with LID was the restoration of iSPN axospinous synapses. Near-complete loss of SNc dopaminergic neurons was accompanied by a significant reduction in dendritic branching and total dendritic arbor length in both dSPNs and iSPNs. The reduction in dendritic length was ~25% in dSPNs and 20% in iSPNs. A similar dendritic atrophy is a common feature of SPNs in PD patients [39] , [40] . Dendritic atrophy was not reversed by L-DOPA administration, suggesting it was not caused by deficits in striatal dopamine release. One factor released by SNc dopaminergic neurons that would be expected to have common effects on dSPNs and iSPNs is the brain-derived neurotrophic factor [41] , [42] . In a number of neurons, the brain-derived neurotrophic factor signalling through TrkB receptors increases dendritic branching and complexity [43] . Given that previous studies with partial lesions did not find dendritic atrophy [21] , it is possible that there is a threshold of dopamine denervation for this phenomenon to occur. Previous work has shown that profound dopamine depletion, mimicking advanced PD, induces a rapid loss of spines and glutamatergic axospinous synapses in iSPNs, but not neighbouring dSPNs [16] . This observation gave a structural foundation for earlier biochemical studies showing that ionotropic glutamate receptors found at these synapses (GluA1, GluN1 and GluN2B) are downregulated by 6-OHDA lesions [44] , [45] , [46] . What was left unresolved by these studies was the origin of the presynaptic terminal pruned. Our work demonstrated that much of this pruning was of corticostriatal axospinous synapses, as their density was reduced by ~40% in iSPNs from parkinsonian mice. This conclusion is consistent with the recent observation that striatal immunoreactivity for cortically expressed vesicular glutamate transporter 1 is downregulated in parkinsonian rats, while the expression of vGlut2 is unaltered [20] . It remains to be determined whether there is concomitant pruning of thalamostriatal axospinous synapses in this rodent model of PD, as seen in other PD models [47] , [48] . In addition to pruning excitatory corticostriatal synapses, iSPNs downregulated their intrinsic excitability in response to 6-OHDA lesions. Both somatic excitability and dendritic excitability fell in iSPNs. The ionic mechanisms underlying this change remain to be determined, but it is clear that they complement the pruning of excitatory synapses to decrease iSPN spiking following dopamine depletion. In contrast to iSPNs, dSPNs did not exhibit any obvious change in axospinous synapse density following induction of the parkinsonian state and the loss of excitatory D 1 R signalling. This finding contrasts with that of Suarez et al. [21] who reported a reduction in dSPN spine density following 6-OHDA lesioning. One potential explanation for the difference is that Suarez et al. [21] used intrastriatal 6-OHDA injections to lesion dopaminergic fibres. Although this approach has several features of relevance to PD, intrastriatal 6-OHDA injections trigger a neuroinflammatory response that might induce nonspecific spine loss [49] , [50] . Why in our model dSPNs exhibited intrinsic but not synaptic homeostatic plasticity is not clear. It is possible that D 1 R signalling, which is lost in the parkinsonian state, is necessary in dSPNs for de novo spine generation [51] . Thus, iSPNs and dSPNs manifested compensatory, cell-specific homeostatic plasticity in the parkinsonian state. These adaptations should diminish the imbalance in the activity of direct and indirect pathway triggered by the loss of dopaminergic signalling. Work in profoundly parkinsonian rats suggests that these homeostatic adaptations are not successful in restoring the balanced excitability seen in the healthy striatum [52] , [53] . However, in early stages of PD, where there still is a substantial dopaminergic innervation of the striatum, the homeostatic mechanisms described here, working in concert with biochemical adaptations described previously [54] , [55] , could help maintain a balance in the average activity of dSPNs and iSPNs. However, not all the changes in SPNs were homeostatic. In addition to changes in intrinsic excitability and synapse number, sustained perturbations in neuronal activity often result in the global up- or downregulation of synaptic strength, a phenomenon referred to as synaptic scaling [56] . Scaling preserves information stored in the relative weights of synaptic connections. Scaling did not occur in the PD models. In iSPNs, where spines were pruned following dopamine depletion, residual synaptic strength was increased—not decreased as expected of a scaling mechanism. In dSPNs, where there was no change in axospinous synapse number, synaptic strength was decreased following dopamine depletion — not increased as expected of a scaling mechanism. These anti-homeostatic adaptations probably reflect the fact that dopamine not only controls intrinsic excitability but also synaptic plasticity [2] . In principle, homeostatic adaptations in SPNs driven by dopamine depletion should be reversed by L-DOPA treatment. This was true in iSPNs. Consistent with recent anatomical work [20] , [21] , [22] , high-dose L-DOPA treatment restored the density of functional axospinous, corticostriatal glutamatergic synapses. Importantly, treatment with a low dose of L-DOPA did not restore iSPN spine deficits. In addition, somatodendritic excitability rose to levels indistinguishable from those of iSPNs in control mice. At face value, these observations suggest that iSPNs were restored to their normal, pre-parkinsonian state. However, there are reasons to doubt this conclusion. First, although our optogenetic experiments demonstrate that high-dose L-DOPA treatment re-established functional corticostriatal connectivity, they do not show whether connectivity with the appropriate cortical regions were re-established. This question is now being pursued using anatomical approaches. Lastly, the fact that only high doses of L-DOPA increased the density of corticostriatal synapses in iSPNs suggests that this adaptation could be linked to the network pathophysiology underlying LID. In dSPNs, L-DOPA treatment partially reversed the changes in intrinsic excitability induced by the parkinsonian state. However, L-DOPA treatment did more than simply reverse depletion-induced adaptations. Most notably, L-DOPA triggered the pruning of corticostriatal axospinous synapses. This adaptation was seen at both low and high doses of L-DOPA, dissociating it from the induction of dyskinesia per se . As mentioned above, in a number of other neurons, sustained perturbations in activity—such as those created by dopamine depletion—result in global synaptic scaling to restore activity to a predetermined set point [56] . With global scaling of synaptic strength, relative synaptic weights sculpted by learning are preserved. Thus, cellular memories stored in synaptic weight are not erased or distorted. However, SPNs did not exhibit this type of synaptic scaling. Instead of scaling synaptic strength, SPNs eliminated axospinous synapses to maintain a stable synaptic input. This could reflect a process similar to what has been described as ‘local’ synaptic homeostatic scaling [57] . Here, activity-dependent potentiation of synapses triggers depression of neighbouring synapses to stabilize regional synaptic weight. This kind of regional homeostatic mechanism might explain the stability of cortical excitation of SPNs in the parkinsonian state seen in our experiments using optogenetic approaches, as well as that seen by others using electrical stimulation in vivo [53] . The situation in dSPNs appears to be more complicated. In the LID model, aggregate cortical synaptic excitation of dSPNs fell, as did spine density and the relative number of strong corticostriatal synapses. Taken at face value, this is inconsistent with the homeostatic model. It also seems inconsistent with work, suggesting that LID is dependent on aberrant strengthening of corticostriatal synapses triggered by the loss of depotentiation in dSPNs [58] . However, there are most likely two phases in the dSPN response to L-DOPA. During the active treatment (‘on’ L-DOPA), D 1 R stimulation could induce synaptic potentiation and an elevation in intrinsic excitability; this could trigger synaptic pruning. After the last L-DOPA dose (when our measurements were taken), striatal dopamine levels fall, pushing down dSPN excitability and enabling depotentiation of strong synaptic connections, shifting the distribution of synaptic amplitudes. The time course of these changes remains to be precisely mapped, but it would appear that the subtraction or addition of spines takes more than the 48 h between L-DOPA injections in our experiments. Although the mechanisms governing the subtraction or addition of axospinous synapses in SPNs are poorly understood, local Ca 2+ signalling could be important. One piece of evidence that is consistent with this conclusion is that the loss of iSPN synapses following dopamine depletion is regulated by Cav 1.3 L-type Ca 2+ channels that are positioned near glutamatergic synapses [16] , [59] . Furthermore, in our studies the abundance of Ca 2+ -permeable extrasynaptic NMDARs was strongly correlated with spine pruning whether in iSPNs or dSPNs. Although it remains to be determined whether they are causally linked to pruning, extrasynaptic NMDARs are coupled to signalling pathways that destabilize spines [60] . The fact that the elevation in extrasynaptic NMDARs was cell type- and state-specific adds an important dimension to previous work correlating their striatal appearance and the pathophysiology of PD [37] . The rapid and bidirectional effects of dopamine on the excitability of iSPNs and dSPNs have dominated basal ganglia models of PD for decades. This spatially diffuse modulation [61] , [62] , [63] serves to globally bias action selection, but it cannot determine precisely what actions are endorsed or vetoed. This function must be determined by the strength and pattern of corticostriatal connections with SPNs. These connections are sculpted by outcome-dependent release of dopamine. This sculpting is presumably what underlies striatal learning. In the severely parkinsonian state, L-DOPA administration continues to shape synaptic strength, but it is shaped in a way that is divorced from the outcome of action selection because it is not arbitrated by dopaminergic neurons [6] , [58] . Moreover, synaptic connectivity in this state is also being sculpted by cell autonomous homeostatic mechanisms that have nothing to do with action selection outcomes. Viewed from this perspective, LID (and the parkinsonian state) can be seen as a manifestation of aberrant striatal learning, not simply an imbalance in direct and indirect pathway activity. Animals Male C57Bl/6 and FVB mice expressing enhanced green fluorescent protein (eGFP) or tdTomato under control of either the Drd1a or Drd2 receptor regulatory elements were used. All the mice used for experimentation were hemizygous for these transgenes [26] . For some experiments, BAC transgenic mice were crossed with a transgenic line expressing ChR2 in the cortex (Thy1-ChR2). All mice were 6–10 weeks of age before stereotaxic surgery and housed under a 12-h light/dark cycle with food and water provided ad libitum throughout the study. Protocols were reviewed and approved by the Northwestern Institutional Animal Care and Use Committee and Malmo-Lund Ethical Committee on Animal Research. Unilateral model of PD and LID Mice were anaesthetized with an isoflurane precision vaporizer (Smiths Medical PM, Inc., Norwell, MA), placed in a stereotaxic frame (David Kopf Instruments, Tujunga, CA) with a Cunningham adaptor (Harvard Apparatus, Holliston, MI) and a hole was drilled over the medial forebrain bundle. After exposing the skull, 3.5 μg of 6-OHDA HCl in 1 μl volume of sterile saline with 0.02% ascorbic was injected using a calibrated glass micropipette (Drummond Scientific Company, Broomall, PA) pulled on a P-97 Sutter Instruments (Novato, CA) at the following coordinates: AP: −0.7, ML: 1.2, DV: −4.75. Sham-operated mice underwent identical surgical procedures and were administered 1 μl of vehicle (saline with 0.02% ascorbic acid) into the medial forebrain bundle. Mice were monitored daily post-op and supplemented with saline injections and high-fat/high-sucrose food as needed based on prior studies [64] . Two weeks post-op, mice underwent a cylinder test ( Supplementary Fig. 1a ) to measure asymmetrical forelimb use to verify the lesion as previously described [64] . In brief, mice were placed in a 600-ml glass beaker for 3 min (subjects were not acclimated to the testing room or beaker) and number of ipsilateral and contralateral (to lesioned hemisphere) forelimb weight bearing paw contacts were counted; data are expressed as % contralateral paw contacts. Within 1–7 days of the cylinder test, mice underwent behavioural testing for abnormal involuntary movements (AIMs; Supplementary Fig. 1b ) as previously described [65] , [66] . In brief, mice were transferred to a behavioural testing room, placed in standard housing cages without bedding and administered intraperitoneal injections. Behavioural testing occurred every other day for a total of five test sessions. Four groups were tested: sham, 6-OHDA lesion, 6-OHDA lesion+low-dose L-DOPA and 6-OHDA lesion+high-dose (dyskinesiogenic) L-DOPA. The low-dose L-DOPA group received 1.0 mg kg −1 L-DOPA (eliciting very mild or no AIMs) for all five test sessions and the high-dose group received 6.0 and 12.0 mg kg −1 L-DOPA for the first two and last three behavioural sessions, respectively. Benserazide was coadministered at 12.0 mg kg −1 with all L-DOPA treatments. AIMs (axial, limb and orolingual movements) were scored as previously described [65] , [66] . In brief, abnormal axial, limb and orolingual behaviours were observed for 1 min every 20 min for a total of 180 min and rated on a scale from 0 to 4 for each parameter; scores of 0 equates no abnormal behaviour, 1 exhibiting abnormal behaviour for less than half of the 1-min observation period, 2 exhibiting abnormal behaviour for more than half of the observation period, 3 abnormal behaviour for the entire observation period but was able to be interrupted and 4 abnormal behaviour for the entire observation period and resistant to interruption. Physiological experiments were performed 1–4 days after the last L-DOPA/saline administration. Striatal and nigral sections from a subset of mice were stained with tyrosine hydroxylase to verify successful lesion. Brain slice preparation Mice were anaesthetized with a mixture of ketamine (50.0 mg kg −1 ) and xylazine (4.5 mg kg −1 ), and transcardially perfused with modified artificial cerebrospinal fluid (aCSF) containing (in mM) 124.0 NaCl, 3.0 KCl, 1.0 CaCl 2 , 2.0 MgCl 2 , 26.0 NaHCO 3 , 1.0 NaH 2 PO 4 and 16.66 glucose, brain removed and 240–275 μm parasagittal slices sectioned. Slices were transferred to a holding chamber and incubated in aCSF containing (in mM) 2.0 CaCl 2 and 1.0 MgCl 2 at 34 °C for at least 30 min, after which the holding chamber was moved to room temperature for electrophysiology experiments. 2PLSM and anatomy iSPNs and dSPNs in the dorsolateral striatum were identified by somatic eGFP and tdTomato, respectively, using 2PLSM with an Ultima Laser Scanning Microscope system (Prairie Technologies, Middleton, WI) or a Zeiss LSM710 NLO with MaiThai laser (Spectra Physics, Santa Clara, CA). A DODT contrast detector system was used to provide a bright-field transmission image in registration with the fluorescent images. The red tdTomato (554–581 nm) and green eGFP (490–560 nm) were acquired with 810 nm excitation using a two-photon laser (Verdi/Mira laser) or 543 nm with a single-photon laser (HeNe). SPNs were patched with video microscopy using either a Hitachi charge-coupled device camera and an Olympus X60/0.9 numerical aperture lens or an Axiocam charge-coupled device camera (Zeiss) and a W Plan-Apochormat 63x/1.0 numerical aperture objective (Zeiss). For anatomical assessments whole-cell images were obtained with 0.389 μm 2 pixels, with 0.5 μm z-steps and sholl’s analysis performed on three-dimensional reconstructions with NeuroLucida (Williston, VT) or Imaris (Bitplane, AG Zurich, Switzerland). High-magnification images of dendritic segments (proximal: <80 μm from soma; distal: >80 μm from soma) were acquired with 0.15 μm 2 pixels with 0.3 μm z-steps. High-magnification images were deconvolved in AutoQant (MediaCybernetics, Rockville, MD) and semi-automated spine counting performed using three-dimensional reconstructions in NeuronStudio (CNIC, Mount Sinai School of Medicine, New York). Total spine estimates were calculated by averaging proximal and distal spine densities for each cell and multiplying by the following: median total dendritic length for treatment group—(30 × median number of primary dendrites for treatment group). Thirty multiplied by the number of primary dendrites was subtracted from the total dendritic length, because the first 30 μm of a primary dendrite are aspiny or have minimal spines. Electrophysiology Patch pipettes were pulled from thick-walled borosilicate glass on a Sutter P-1000 puller. Pipette resistance was typically 3–4.5 MΩ when filled with recording solution. The internal recording solutions contained (in mM) 135.0 KMeSO 4 , 5.0 KCL, 0.16 CaCl 2 , 10.0 HEPES, 2.0 Mg-ATP, 0.5 Na-GTP, 5 phosphocreatine-Tris, 5.0 phospocreatine-NA and 0.1 spermine or 120.0 CsMeSO 3 , 5.0 NaCl, 0.16 CaCl 2 , 10.0 TEA-CL (tetraethylammonium-Cl), 10.0 HEPES, 5.0 QX-314, 4.0 Mg-ATP, 0.3 Na-GTP, or 130.0 CsMeSO 3 , 5.0 HEPES, 0.25 EGTA, 10.0 Phosphocreatine-di(Na), 2.0 ATP-Mg, 0.5 GTP-Na, 5.0 TEA-Cl, 1.0 QX-314; pH was adjusted to 7.25–7.30 and osmolarity 270–280 mosM. In experiments involving two-photon microscopy, the internal recording solution lacked CaCl 2 and 50 μM Alexa Fluor 568 hydrazide sodium salt was added for visualization of cells and 200 μM Fluo-4 pentapotassium to detect calcium signals. Slices were continuously perfused with carbogen (95% O 2 ; 5% CO 2 )-bubbled aCSF. For whole-cell recordings, slices were transferred to a submersion-style recording chamber mounted on an Olympus BX51 upright, fixed-stage microscope or on a Zeiss LSM 710 NLO; once whole-cell configuration was achieved the internal solution was allowed to equilibrate for at least 15 min before beginning experiments. Electrophysiological recordings were obtained using a Multiclamp 700 A or 700B amplifier with stimulation and display obtained as previously described [25] with custom-written shareware package Winfluor (John Dempster, Strathclyde Universty, Glasgow, UK), which automates and synchronizes the two-photon imaging and electrophysiological protocols or pClamp (Molecular Devices, Inc., Sunnyvale, CA). The amplifier bridge circuit was adjusted to compensate for serial resistance and monitored throughout the experiment. Recordings were performed at room temperature and filtered at 1–2 kHz. Intrinsic excitability was assessed in current clamp with 500 ms somatic current injection. Synaptic NMDA/AMPA ratios were determined in voltage clamp with a Cs + -based internal solution and aCSF supplemented with 10.0 μM glycine, 50.0 μM picrotoxin and 1.0 μM tetrodotoxin (TTX). Spines were visualized and somatic responses to glutamate uncaging at spines was tested with cells held at −70 mV (AMPA component) and at +40 mV (NMDA component). Stimulation was performed on four to five spines per dendritic segment, with 1.5 s between each spine stimulation. Stimulation at each voltage level was repeated three times and responses were averaged. Uncaging was performed as previously described [67] ; MNI glutamate (5 mM; Tocris Cookson) was superfused at 0.4 ml h −1 and uncaged using 1 ms pulses of 720 nm light, controlled by a third Pockels cell modulator (model 302, Con Optics) and typically about 15 mW in strength. Photolysis was adjusted to closely mimic spontaneously occurring AMPA EPSCs. To complement and expand the findings using uncaging techniques, neurons from Thy1-ChR2-D2 eGFP and Thy1-ChR2-D1 tdTomato were patched with a Cs + -based internal solution and ChR2 was stimulated with 473 nm light using a blue LED (full-field stimulation) to excite all cortical afferents (CoolLED, Yorktown Heights, NY); light intensity was calibrated to ~150 pA response with cells held at −70 mV. Similar to uncaging studies, the AMPA component and NMDA components were measured with cells held at −70 and +40 mV, respectively, in optogenetic experiments. For all NMDA/AMPA assessments, NMDA component was measured 50 ms after the peak to minimize potential contamination by AMPA currents. To further assess synaptic properties, corticostriatal AMPA-mediated mEPSCs were assessed by asynchronous release achieved by substituting Ca 2+ with Sr 2+ as previously described [34] , and electrically stimulating between layers V and VI in the motor cortex with a parallel bipolar electrode (Frederick Haer & Co., Bowdoin, ME). StrEPSCs were collected during a 300-ms period beginning 50 ms after each electrical stimulation (delivered once every 15 s) in the presence of 10.0 μM SR 95531 (gabazine) and 10.0 μM (R)-CPP. Miniature events were analysed using Minianalysis software (Synaptosoft, Decatur, GA) with detection parameters set at >5 pA amplitude and individually verified. For analysis of each cell, between 50 and 100 sweeps were used. Access resistance was continuously measured and experiments were rejected if it changed significantly. Channelrhodopsin-assisted circuit mapping Cells from Thy1-ChR2-D2 eGFP were patched with a Cs + -based internal solution with 100 μM 4.0 AP, 1.0 μM TTX, 10.0 μM Gabazine and 1.0 μM CGP 35348 added to aCSF. Input–output curves were generated using full-field illumination (473 nm light; CoolLED) from 10%-80% LED power at 10% steps in voltage clamp; each LED intensity was repeated three times at 10-s intervals and data presented as average EPSC amplitude. For corticostriatal axospinous, circuit mapping proximal (<80 μm from the soma) and distal (>80 μm from the soma) were identified, and a Prairie Instruments blue laser (473 nm) was targeted adjacent to a spine in voltage clamp with minimal fixed diameter (~1 μm); 6–10 spines were sampled per dendritic segment. Laser intensity was calibrated to the minimum laser power to elicit at least one synaptic response from the series of spines; this minimum threshold was then doubled for circuit mapping. Synaptic responses were recorded six times at 10-s intervals and data presented as the average response. Statistics Data analysis was performed with Clampfit9.2 (Molecular Devices, Inc.), Igor Pro 5.0 (WaveMetrics, Lake Oswego, OR), Matlab R2009b (Mathworks, Natick, MA), and Minianalysis software (Synaptosoft). Statistical analyses were performed using Sigmastat 3.5 (Systat Software Inc., San Jose, CA) and Prism 5 (GraphPad, La Jolla, CA). Data are reported as average±s.e.m. or box and whisker plots showing median, quartiles and range. Statistical evaluations were performed using non-parametric Mann–Whitney U -test of significance, Kruskal–Wallis non-parametric test with Dunns post-hoc and two-way analyses of variance with Newman–Keuls post-hoc where appropriate. Differences were considered significant if P <0.05. How to cite this article: Fieblinger, T. et al. Cell type-specific plasticity of striatal projection neurons in parkinsonism and L-DOPA-induced dyskinesia. Nat. Commun. 5:5316 doi: 10.1038/ncomms6316 (2014).